Niche and host-associated functional signatures of the root surface microbiome Plant microbiomes are critical to host adaptation and impact plant productivity and health. Root-associated microbiomes vary by soil and host genotype, but the contribution of these factors to community structure and metabolic potential has not been fully addressed. Here we characterize root microbial communities of two disparate agricultural crops grown in the same natural soil in a controlled and replicated experimental system. Metagenomic (genetic potential) analysis identifies a core set of functional genes associated with root colonization in both plant hosts, and metatranscriptomic (functional expression) analysis revealed that most genes enriched in the root zones are expressed. Root colonization requires multiple functional capabilities, and these capabilities are enriched at the community level. Differences between the root-associated microbial communities from different plants are observed at the genus or species level, and are related to root-zone environmental factors. The holobiont paradigm, first introduced at the late 20th century [1] , identified the microbiota associated with macro-organisms as an auxiliary arsenal of genetic material, acting as an integrated functional unit [2] . The ubiquity of such interactions and their extensive effect on host adaptation has been recognized by plant scientists for over a century [3] , [4] . Case studies, including mycorrhiza and legume-rhizobium symbiosis, have been extensively examined at the functional and molecular level. The analysis of complex plant-associated microbial communities, such as those naturally assembling on plant roots, however, has been fundamentally limited by technical constraints and sequencing depth. Recently developed high-throughput sequencing technologies have facilitated comprehensive surveys of host-associated microbiomes. In addition to providing a census of microbial taxonomic diversity, such data have enabled the characterization of genomic elements related to host colonization and their function. Recent studies of the commensal microbiome of human and other mammals have revealed broad-scale and highly profound effects on host physiology. These studies have demonstrated strong linkages between mammalian microbiome structure and environmental factors [5] , diseases [6] and even the functioning of the host neural system [7] . The integral role of the commensal microbiome of plants on host physiology, phenology, development and fecundity has been extensively described [4] . Specifically, plant root microbiomes vary by soil type and host genotype [8] , [9] , [10] and greatly impact plant productivity [11] , health [3] and ecosystem services such as phytoremediation [12] and carbon sequestration [13] . The elucidation of the microbiome functional characteristics, as a key to assess the potential and actual effect on the plant host, however, was rendered highly challenging due to the enormous taxonomic and genetic complexity of the microbial community [3] . Indeed, microbiome-level functional studies that aim for the generalization of successful root colonization mechanisms have not yet been reported. In this study, we examined the genetic and taxonomic composition, and gene expression patterns (function) of root surface (that is, rhizoplane) microbial communities of two important but highly different crop plants, wheat and cucumber. We describe bacterial genetic determinants linked to plant host colonization and root dominance. Genes and pathways, including those coding for degradation of plant polysaccharides, two-component systems, secretion systems and lipopolysaccharide biosynthesis, were enriched in the root metagenomes. The functional metagenomic profiles of root-associated bacterial communities of both plant hosts were highly similar. Yet, communities of the two plant hosts were distinguished by host-specific enrichment of taxa, as well as by unique expression patterns of many genes, particularly those related to environmental conditions and stressors. Combined analysis of metagenome and metatranscriptome data enabled discrimination of two microbial community assembly processes: a general, non-host-specific, but reproducible root community functional selection in response to the global nature of the habitat (that is, rhizosphere effect), and taxon-specific selection based on functional response to the specific host phenotype. Soil-root gene catalogue and phylogenetic analysis Our metagenomic data were collected from a biologically replicated experiment, conducted under controlled conditions, to minimize sources of environmental variation. Wheat ( Triticum turgidum ) and cucumber ( Cucumis sativus ) roots were collected from 12-day-old seedlings, corresponding to first true leaf extension for both plant species. Genomic DNA (gDNA) of rhizoplane communities (RC) was extracted from root samples (three independent replicates for each plant species) and respective soil samples (two independent replicates for each plant species), using standard procedures [14] . 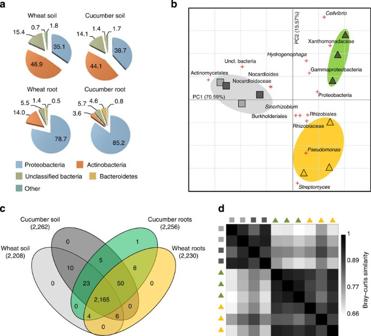Figure 1: Taxonomic and functional characterization of soil and rhizoplane bacterial communities. (a) Pie charts of the taxonomic annotation of bacterial metagenomic sequence reads among dominant phyla. Numbers indicate mean relative abundance (n=2 for soil samples,n=3 for rhizoplane samples) as a percentage of total, based on rarefaction to 5 million reads per sample. (b) Bi-plot of principal component (PC) analysis of bacterial community composition, based on covariance matrix derived from the metagenome analysis. Numbers in parenthesis indicate the percentage of variance explained by each PC. Light grey square, wheat soil; dark grey square, cucumber soil; orange triangle, wheat roots; green triangle, cucumber roots; red cross, factor coordinates of taxa with highest contribution to variation in the first and second PCs. (c) Venn diagram depicting numbers of KEGG orthology (KO) groups detected in soil and root metagenomes of wheat and cucumber. Numbers in parentheses indicate the total number of KOs detected within denoted samples. (d) Heat map showing similarity of KO profiles between samples. Pair-wise Bray–Curtis similarities were calculated from the trimmed means ofM-values method (TMM)-normalized read counts of KO group profiles. Uncl. bacteria, unclassified bacteria. Shotgun DNA libraries generated from these gDNA samples were sequenced on an Illumina HiSeq2000 instrument, and in total, 87.6 gigabases (Gb) of paired-end sequence data were generated, with an average of 43.8 million paired reads per sample ( Supplementary Table 1 ). De novo assembly of the sequence data was performed to create a non-redundant gene catalogue from soil and RC. The total length of the non-redundant assembly was 532.6 megabases (average contig length 269 bp, range: 101 to 49,612 bases) from which ~2.4 million partial genes with an average length of 228 bases were predicted. Our gene catalogue was used for alignment of individual metagenome sequence reads, and represented 34.2±6.1% of soil reads, 70.8±10.3% of cucumber RC reads and 49.2±8.7% of wheat RC reads ( Supplementary Table 1 ), indicative of the higher microbial and genetic diversity present in the soil. To determine the taxonomic affiliation and putative function of the predicted genes, a translating BLAST (BLASTX) [15] alignment was performed against the NCBI non-redundant database and the lowest common ancestor (LCA) was determined using Metagenome Analyzer (MEGAN), down to the species level ( Supplementary Fig. 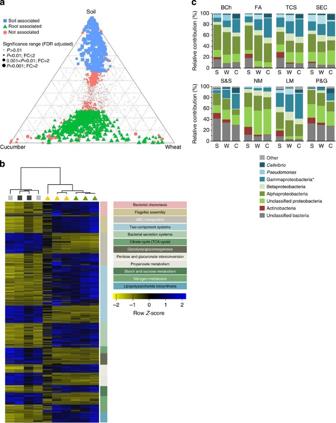Figure 2: Profiles of soil and rhizoplane bacterial community functional potential. (a) Ternary plot where each symbol represents a KO group identified in soil or rhizoplane metagenomes. The position of each symbol is determined by the contribution of the indicated samples to the total normalized read count for the specific KO. The size of the symbol indicates the FDR-adjustedPvalue in an edgeR differential abundance test. The dashed grid inside the plot indicates 10% increments of contribution from each sample type. (b) Pathways with the greatest significant differential abundance (DA) of KOs. Shown are relative abundances of differentially abundant KOs, normalized byZ-score across all data sets. UPGMA clustering of samples (top) is based on Spearman correlations. Light grey square, wheat soil (n=2); dark grey square, cucumber soil (n=2); orange triangle, wheat roots (n=3); green triangle, cucumber roots (n=3). (c) Relative contribution of different taxonomic groups to root-enriched genes within key root-enriched pathways. Relative contribution is presented as average percent of the total reads assigned to root-enriched genes within a functional class. C, cucumber; S, soil; W, wheat; BCh, bacterial chemotaxis; FA, flagellar assembly; LM, lipopolysaccharide metabolism; NM, nitrogen metabolism; P&G, pentose and glucuronate interconversion; SEC, bacterial secretion systems; S&S, starch and sucrose metabolism; TCS, two-component systems. *excludingPseudomonasandCellvibrio. 1 ; Supplementary Table 2 ). To compare the genetic composition of communities and abundances of bacterial taxa between root and soil communities, sequence dataset sizes were equalized by random sub-sampling of five million reads from each sample (total 50 million reads; Supplementary Data 1 ). At a coarse phylogenetic level (phylum-level), soil microbial communities were highly similar to each other, as were RC, while RC and soil communities diverged significantly ( Fig. 1a ). The RCs were dominated by proteobacteria (78.7–85.2% of reads); whereas in the soil, proteobacteria represented a significantly smaller proportion of the community (35.1–38.7% of reads) (Mann–Whitney U -test, P <0.05). The most salient shift was an increase in relative abundance of Gammaproteobacteria (from 5.1% in soil to 25.2% in RC). The relative abundance of Alphaproteobacteria, the dominant class of RC bacteria (38.1% of the total bacterial reads) was significantly higher (by 1.5-fold) in root than soil (Mann–Whitney U -test, P <0.05). Actinobacteria, abundant in the soil (44.1–46.9% of reads), were minor components of RCs (3.6–14.0% of reads; Fig. 1a ). At a finer taxonomic resolution, the soil and RC metagenomes were grouped using principal component analysis into three distinct clusters, consisting of soil samples from both plant systems, cucumber RC and wheat RC ( Fig. 1b ). The first principal component (PC) represented 70.6% of the variance and was correlated with niche (soil versus root). The second PC represented 15.6% of the variance and was correlated with host plant. Thus, consistent with prior findings based on 16S rRNA gene amplicon sequencing [14] , these data demonstrate that the niche produces the strongest differentiation in microbial community, but host type also provides for significant differentiation of the rhizoplane microbiome. 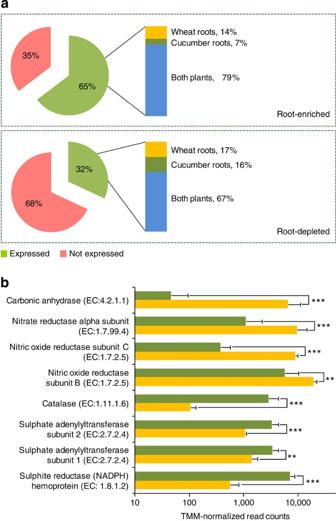Figure 3: Expression analysis of wheat and cucumber rhizoplane bacterial communities. (a) Expression of genes belonging to root-enriched and root-depleted KO groups identified in the metagenome gene catalogue. Frequencies (%) are presented. green section, expressed; pink section, not expressed. (b) Representative key genes (top 10% expression level) differentially expressed between wheat (n=3) and cucumber (n=3) rhizoplane bacterial communities (green=cucumber, yellow=wheat). Mean±standard deviation of TMM-normalized read counts are presented. ** FDR<0.01; *** FDR<0.001, edgeR differential expression test. The taxonomic groups with highest loadings on the 1st and 2nd PCs were among the most dominant groups, and their abundances differed significantly according to niche and host ( Supplementary Table 3 ). For example, sequences derived from bacteria of the genera Cellvibrio and Pseudomonas (both Gammaproteobacteria from the family Pseudomonaceae), both contributing to the 2nd PC, were respectively abundant in RC of cucumber (8.24%) and RC of wheat (6.27%), but present at low abundance in the respective soils (0.74 and 0.37%). These results are in agreement with previous 16S rRNA gene surveys of several plant systems [9] , [14] , [16] , [17] , indicating robust specificity of association between plant host and microorganisms. Figure 1: Taxonomic and functional characterization of soil and rhizoplane bacterial communities. ( a ) Pie charts of the taxonomic annotation of bacterial metagenomic sequence reads among dominant phyla. Numbers indicate mean relative abundance ( n =2 for soil samples, n =3 for rhizoplane samples) as a percentage of total, based on rarefaction to 5 million reads per sample. ( b ) Bi-plot of principal component (PC) analysis of bacterial community composition, based on covariance matrix derived from the metagenome analysis. Numbers in parenthesis indicate the percentage of variance explained by each PC. Light grey square, wheat soil; dark grey square, cucumber soil; orange triangle, wheat roots; green triangle, cucumber roots; red cross, factor coordinates of taxa with highest contribution to variation in the first and second PCs. ( c ) Venn diagram depicting numbers of KEGG orthology (KO) groups detected in soil and root metagenomes of wheat and cucumber. Numbers in parentheses indicate the total number of KOs detected within denoted samples. ( d ) Heat map showing similarity of KO profiles between samples. Pair-wise Bray–Curtis similarities were calculated from the trimmed means of M -values method (TMM)-normalized read counts of KO group profiles. Uncl. bacteria, unclassified bacteria. Full size image Functional genomics of rhizoplane versus soil communities To obtain insight into the physiological capabilities of the microbial communities, and to link taxonomic shifts with functional shifts driving niche- and host- differentiation, we performed a functional characterization of the metagenomes. All the bacterial genes in our metagenome gene catalogue were annotated using the KEGG database [18] to assign putative functions. 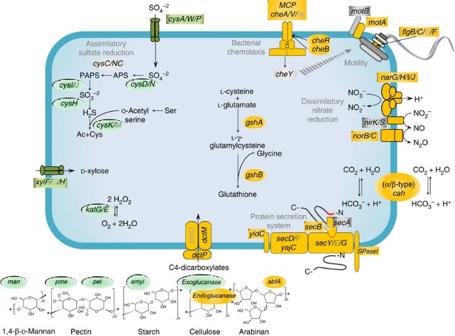Figure 4: Schematic overview of host-related variation in gene expression of rhizoplane microbiomes. Genes highlighted in orange (involved in bacterial chemotaxis, flagellar assembly, denitrification, glutathione synthesis, protein export and C4-dicarboxylates transport) were more abundantly expressed in the wheat RC. Genes highlighted in green (encoding for enzymes for sulphate uptake, assimilatory sulphate reduction, plant cell-wall polysaccharide degradation, enzymes, xylose uptake and catalase) were more abundantly expressed in the cucumber RC. In total, 2,351 different bacterial KEGG orthologs (KOs) were detected, and 41.6±3.6% of bacterial sequences that aligned to the gene catalogue were assigned to a KO category ( Supplementary Table 4 ). After filtering out KOs with extremely low total abundance (three reads per million or fewer) and normalization of the data using the trimmed means of M -values method [19] , the soil and RC functional profiles were collectively comprised of 2,272 KOs ( Supplementary Data 2 ). Based solely on presence, the majority of identified functional attributes (2,165 KOs) were shared between soil and RC assemblies ( Fig. 1c ). Indeed, as root-associated microbial communities were derived from the same soil pool, this result should be expected, provided that a sufficient depth of coverage of the community metagenome was achieved. Although sharing the vast majority of KOs, the functional profiles of RC and soil bacterial communities were significantly discriminated based on the relative abundance of individual KOs in each sample ( Fig. 1d , analysis of similarities with 10,000 permutations, based on Bray–Curtis similarities P <0.01, R =0.9603). The relative abundance data were used to screen for KOs significantly enriched or depleted in the RC metagenomes compared with the soil metagenomes using the edgeR [19] , [20] and SAMseq software packages [21] . Under the criteria chosen (fold change >2, false discovery rate (FDR)-adjusted P value <0.01 and q value <0.001), 787 KOs (34.6% of total) were differentially abundant (DA) in root communities compared with the soil community metagenomes, with 424 KOs enriched (18.6%) and 363 depleted (16.0%; Fig. 2a ; Supplementary Data 3 ). The relationship between relative abundance of genes in metagenomes and their differential abundance in the soil and root environment was examined. The most abundant KOs (>10,000 reads in total) had a lower frequency of significant differential abundance between soil and root when compared with KOs of lesser overall abundance ( χ 2 test, P <0.001; Supplementary Fig. 2 ). Thus, the most abundant KOs were not niche specific, but represented genes involved in central pathways found in many organisms. In addition, we observed multiple pathways in which relatively high proportions of the KOs within that pathway were DA ( Supplementary Table 5 ). For example, of the 20 KOs representing the lipopolysaccharide biosynthesis pathway, 16 (80%) were significantly more abundant in the RC metagenomes. The pathways showing highest rates of DA (greater than 20% of KOs within the pathway) are depicted in Fig. 2b . Figure 2: Profiles of soil and rhizoplane bacterial community functional potential. ( a ) Ternary plot where each symbol represents a KO group identified in soil or rhizoplane metagenomes. The position of each symbol is determined by the contribution of the indicated samples to the total normalized read count for the specific KO. The size of the symbol indicates the FDR-adjusted P value in an edgeR differential abundance test. The dashed grid inside the plot indicates 10% increments of contribution from each sample type. ( b ) Pathways with the greatest significant differential abundance (DA) of KOs. Shown are relative abundances of differentially abundant KOs, normalized by Z -score across all data sets. UPGMA clustering of samples (top) is based on Spearman correlations. Light grey square, wheat soil ( n =2); dark grey square, cucumber soil ( n =2); orange triangle, wheat roots ( n =3); green triangle, cucumber roots ( n =3). ( c ) Relative contribution of different taxonomic groups to root-enriched genes within key root-enriched pathways. Relative contribution is presented as average percent of the total reads assigned to root-enriched genes within a functional class. C, cucumber; S, soil; W, wheat; BCh, bacterial chemotaxis; FA, flagellar assembly; LM, lipopolysaccharide metabolism; NM, nitrogen metabolism; P&G, pentose and glucuronate interconversion; SEC, bacterial secretion systems; S&S, starch and sucrose metabolism; TCS, two-component systems. *excluding Pseudomonas and Cellvibrio . Full size image Analysis of the differential abundance of KOs identified the key genotypic features of root-colonizing bacteria ( Fig. 2b ; Supplementary Data 3 ). The DA analysis identified root-associated enrichment of genes linked to motility (via flagella and twitching), chemotaxis, lipopolysaccharide biosynthesis and plant cell wall polysaccharide-degrading enzymes, particularly cellulose (EC3.2.1.4; EC3.2.1.91), pectin (EC3.1.1.11; EC4.2.2.2), xylan (EC3.2.1.37), mannan (EC3.2.1.78), glucan (EC3.2.1.39) and arabinan (EC3.2.1.55). Genes for aerobic-C4-dicarboxylate sensing and transport ( dct genes), secretion systems types II, III and type VI and quorum sensing systems ( qseC/B -like and rpfC/rpfG -like systems) were also enriched in the RC metagenome. To determine if these gene enrichment/depletion patterns correspond with gene usage in the root niche, we performed a metatranscriptomic analysis of the RC of both plant species. Total RNA was extracted from plant roots (three independent replicates for each plant species), grown under identical conditions as those plants used in the metagenome analysis. Following rRNA depletion and double-stranded cDNA synthesis, sequence libraries were generated, and sequencing was performed on an Illumina HiSeq2000 instrument. The RNA-derived reads were aligned to our gene catalogue and assigned to specific KOs ( Supplementary Tables 1 and 4 and Supplementary Data 4 ). We detected the expression of 274 out of 424 (~65%) root-enriched KOs in the RC metatranscriptome ( Fig. 3a ). Reciprocally, the majority (~68%) of KOs depleted in the RC metagenomes were not detected in the respective metatranscriptomes ( Fig. 3a ). Figure 3: Expression analysis of wheat and cucumber rhizoplane bacterial communities. ( a ) Expression of genes belonging to root-enriched and root-depleted KO groups identified in the metagenome gene catalogue. Frequencies (%) are presented. green section, expressed; pink section, not expressed. ( b ) Representative key genes (top 10% expression level) differentially expressed between wheat ( n =3) and cucumber ( n =3) rhizoplane bacterial communities (green=cucumber, yellow=wheat). Mean±standard deviation of TMM-normalized read counts are presented. ** FDR<0.01; *** FDR<0.001, edgeR differential expression test. Full size image Host impact on functional assembly While host-specific enrichment of taxa was robust ( Fig. 1a ), bacterial communities associated with both plant hosts exhibited similar genetic functional profiles ( Fig. 2a ; Supplementary Data 5 ). In total, only 2.7% of the KOs were differentially abundant between wheat and cucumber root metagenomes. This taxonomic specificity remains to be explained at the functional level. Therefore, the contribution of different taxa to KOs enriched in the two RCs was examined. The relative contribution of proteobacterial open reading frames (ORFs) to these RC-enriched KOs was high both in soil communities and in RC (mean percentage 74.1 and 86.1, respectively). More specifically, among eight KEGG pathways strongly enriched in RCs, the gene pool was dominated by genes from Alpha- and Gammaproteobacteria ( Fig. 2c ; Supplementary Data 6 ). Similarity percentage analysis determined that Pseudomonas and Cellvibrio were the primary taxa responsible for differences between the two host species. Furthermore, in two out of the eight pathways (pentose and glucuronate interconversion and starch and sucrose metabolism; Fig. 2c ), the contribution of Pseudomonas was particularly low, while that of Cellvibrio was high. In these two pathways, nine enzymes were specific to Cellvibrio and were involved in the degradation of glucans (EC:3.2.1.91; EC:3.2.1.39; EC:3.2.1.4; EC:3.2.1.21), and degradation of pectin and further conversion of its metabolites (EC:3.1.1.11; EC:4.2.2.2; EC:4.2.1.7; EC:5.3.1.12; EC:1.1.1.57). In addition to those, genes encoding for mannan (EC:3.2.1.78), arabinan (EC:3.2.1.55) and chitin (EC:3.2.1.14; EC:3.2.1.52), modifying enzymes from Cellvibrio but not from Pseudomonas were detected in the RC metagenomes ( Supplementary Data 7 ). With respect to gene usage, expression of all but one of these 13 enzymes (EC:3.2.1.39) was verified. To assess whether such genes may be involved in host-specific enrichment, differential expression (DE) between the metatranscriptomes was examined. The methods for DE analysis were identical to those used for comparative metagenomic analysis described above. Significantly higher expression of genes encoding mannan and pectin degradation enzymes in cucumber RC relative to wheat RC was verified ( Supplementary Data 8 ). Gene expression patterns reveal host impact A global analysis of DE of bacterial functional genes between the two hosts using KO patterns produced from the metatranscriptomic data was performed. In total, significant DE was confirmed for 238 out of 1,401 expressed bacterial KOs (17.0%). Of these, 97 KOs were more abundantly expressed in cucumber root communities and 141 KOs were more abundantly expressed in wheat RCs ( Supplementary Data 8 ; Supplementary Fig. 3 ). In contrast to the pattern observed for DA genes in the metagenome analysis, even among the top 10% most abundantly expressed KOs, significant DE between wheat and cucumber roots was found, with fold change values as high as two orders of magnitude ( Fig. 3b ). Overall, the functional divergence between the two plant hosts involved many aspects of microbial metabolism and environmental information processing. The central functional variations are illustrated in a schematic diagram ( Fig. 4 ). Examination of the taxa contributing to host differential DE functions revealed that the expression of these genes was not restricted to those taxa that were host-enriched ( Supplementary Table 6 ), indicating that differential expression of genes reflects a host-related physiological adaptation of multiple rhizoplane community members. Some taxa in particular had strong host-specificity, and contributed disproportionally to the pool of differentially expressed genes in the rhizoplane of a single host. For example, the relative contribution of Pseudomonas to DE in wheat was substantial and included 90 of the 141 genes (63.8%) that were more abundantly expressed in wheat RC. Figure 4: Schematic overview of host-related variation in gene expression of rhizoplane microbiomes. Genes highlighted in orange (involved in bacterial chemotaxis, flagellar assembly, denitrification, glutathione synthesis, protein export and C4-dicarboxylates transport) were more abundantly expressed in the wheat RC. Genes highlighted in green (encoding for enzymes for sulphate uptake, assimilatory sulphate reduction, plant cell-wall polysaccharide degradation, enzymes, xylose uptake and catalase) were more abundantly expressed in the cucumber RC. Full size image Among the genes with the most divergent expression patterns between the two plant RCs were those encoding for enzymes of the dissimilatory nitrate reduction pathway ( Fig. 4 ; Supplementary Data 8 ). Specifically, expression levels of respiratory nitrate reductase ( narG/H/I/J ) and nitric oxide reductase ( norB/C ) genes were significantly higher in wheat root samples than cucumber root samples ( P <0.01). Conversely, a significantly higher level of catalase expression (EC:1.11.1.6; EC:1.11.1.21) was observed in the cucumber RC. Furthermore, the cucumber RC had higher relative expression of genes for degradation of a range of plant cell wall-derived polysaccharides, and a high level of expression of genes involved in sulphate uptake and assimilatory reduction ( Figs 3b and 4 ). Root surface colonizing microbial communities are enriched from soil communities. In this study we show that this enrichment process selects for microorganisms with specific physiological capabilities including motility and chemotaxis, polysaccharide degradation, various two-component systems and multiple secretion systems ( Fig. 2b ; Supplementary Data 3 ). Many of these features have been previously individually implicated in bacterial root competence of cultivated model organisms [4] , [22] , [23] . Therefore, our metagenomic study of soil and natural rhizoplane assemblies incorporates and extends prior findings by defining a generalized genetic tool set associated with organisms abundant in root-associated microbial communities independent of host phenotype. Critically, functional capabilities enriched in root systems and detected in root metagenomes are largely expressed and detectable in metatranscriptomes ( Fig. 3a ; Supplementary Data 4 ). Thus, these data confirm that the root selection leads to expression of DA genes. The ‘rhizosphere effect’ is strongest directly at the root surface, and differences between gene abundance and expression patterns between rhizoplane and rhizosphere communities may be observed, as the influence of the soil organic matter is greater in the rhizosphere. While differences in niche properties between the rhizoplane and rhizosphere soil are essential, many of the enriched attributes are shared. Recently, functional attributes of bacterial communities in the rhizosphere soil of soybean were described [24] , and consistent with our study, identified the importance of membrane transport systems and nitrogen metabolism. Conversely, plant cell wall polysaccharide-degrading enzymes, which were key features of rhizoplane bacteria in our study, were not indicated to have a key role in rhizosphere soil community function. As wheat and cucumber are representatives of highly divergent plant lineages (that is, mono- and dicotyledonous plants, respectively), the finding of high congruence demonstrates high overall genetic functional redundancy among bacterial communities associated with distinct hosts. Similarly, in a metagenomic study performed on Ulva australis (marine alga) microbiome, functional similarity rather than taxonomic relatedness was observed to govern epiphytic assembly [25] . Environmental resources provided by the two plant hosts in this study were distinct, however, and ultimately supported enrichment of different taxa ( Fig. 1b ). Wheat and cucumber roots strongly enriched Pseudomonas and Cellvibrio, respectively, in agreement with previous reports [14] , [26] . Careful examination of genes associated with each group revealed that while Cellvibrio retain an array of genes for cell wall polysaccharide degradation, very few such genes were linked to bacteria from the genus Pseudomonas ( Supplementary Data 7 ). In particular, bacteria from the genus Cellvibrio harboured and expressed genes for degradation of pectin and mannan, and these genes were significantly more abundantly expressed in cucumber RC than the wheat RC. Pectin content differs considerably between monocots and dicots and has been reported to be twice as high in cucumber than wheat [27] . Hence, association between measured host-specific properties, and response of the bacterial community, in terms of gene expression and enrichment of specific populations, was observed. Gene expression patterns more strongly discriminated between RCs of the two plants than metagenomic functional profiling, reflecting the divergent phenotypes of these hosts. For example, one of the most striking differences in gene expression patterns between cucumber and wheat RC communities was the high divergence in expression of dissimilatory nitrate reduction genes ( Fig. 4 ; Supplementary Data 7 ). Activation of these denitrification mechanisms implies significant divergence in levels of oxygen availability between the roots of the two plant species, and the presence of nitric oxide (an important environmental stressor and signalling molecule for both plant and bacteria [28] , [29] ) in the wheat root zone. Dissimilatory nitrate reduction has been suggested as a mechanism of rhizosphere competence for bacteria colonizing the root of cereals, and has been tested with Pseudomonas model systems, though the effect is not consistent across multiple plant-microbial systems [30] , [31] . Conversely, high levels of catalase expression in cucumber RC are indicative of the presence of aerobic conditions and excess hydrogen peroxide (H 2 O 2 ) in the cucumber rhizoplane. Prior studies have suggested that H 2 O 2 serves as an important signalling molecule in adventitious root development in cucumber seedlings [32] . Therefore, catalase activity of rhizoplane bacteria may serve as a stress response and as a means to modulate host root development. Gene expression patterns further indicated nutritional differences between RCs of cucumber and wheat; the former more abundantly express a wide variety of cell wall polysaccharide-degrading enzymes, whereas RCs of the latter more abundantly express genes related to C4-dicarboxylate utilization. This suggests differences in the availability of these carbohydrates between hosts. Metagenomic and metatranscriptomic data are required in tandem to elucidate plant-microbial interactions in the near root zone. Here we demonstrate that a suite of broad physiological capabilities such as motility are required for root colonization by bacteria, but that plant–host-species selectivity is more closely related to specific metabolic activities, including polysaccharide degradation and anaerobic respiration. The data generated here provide a comprehensive framework for understanding plant root colonization and plant-mediated selection of taxa, and will serve to guide future plant microbiome research to improve plant health and yield. Plant species and growth conditions The experiment was conducted at the Agriculture Research Organization of Israel, Bet Dagan, Israel during May 2011. Cucumber ( Cucumis sativus , cv. Kfir-413) and wheat ( Triticum turgidum , cv. Negev) were cultivated in sandy loam soil (81% sand, 6% silt and 13% clay) obtained from Maon region, Israel. The dry soil was mixed with Hoagland nutrient solution (6 mM KNO 3 ; 4 mM Ca(NO 3 ) 2 ·4 H 2 O; 2 mM MgSO 4 ·7 H 2 O; 1 mM (NH 4 ) 2 PO 4 ; 50 μM KCl, 25 μM H 3 BO 3 ; 2 μM MnSO 4 ·H 2 O; 2 μM ZnSO 4 ·7 H 2 O; 0.3 μM CuSO 4 ·5 H 2 O; 0.5 μM H 2 MoO 4 , 20 μM Fe-EDTA) at a rate of 1 litre per 3 kg of soil. Seeds were surface-sterilized by soaking in 3% sodium hypochlorite for 1.5 min followed by 70% ethanol for 1.5 min, and were washed three times with sterile water. This procedure was performed to eliminate seed-borne pathogens. The wet sand was distributed into 200 ml plastic pots with four seeds in each. Pots were arranged randomly in a growth chamber and the plants were grown there at 30 °C, with 18 h of daylight. Plants were watered daily with half-strength Hoagland nutrient solution. Plants were grown for 12 days, corresponding to first true leaf extension for both plant species. At this stage, the root systems of both plants were vital along almost the entire root lengths and were approximately the same wet weight per replicate. Sampling of plant and soil material Plants were harvested from six independent pots for each plant species, and the four seedlings in each pot were treated together. Plants were carefully removed with intact roots, and the soil was removed by shaking. To remove loosely adhering particles, roots were immersed in 30 ml of sterile saline (0.85% NaCl) and vortexed at maximum speed for 30 s. This step was repeated with fresh sterile saline, and then roots were blotted on sterile filter paper, quick-frozen in liquid nitrogen and then stored at −80 °C until further use. To minimize effect of sampling procedure on mRNA profile, the procedure was carried out sample by sample and as rapidly as possible (average of 4 min per sample). Bulk soil samples (not root adhering) were taken from each pot (80 g from each pot). Ten grams were quick-frozen in liquid nitrogen and then stored at −80°C until further use, and 50 g were used for analysis of soil chemical properties ( Supplementary Data 9 ). DNA and RNA isolation For each plant species, two replicates of soil and three replicates of root samples were used for genomic DNA extraction. Three additional independent replicates per plant species were used for total RNA extraction from roots. All samples were thawed on ice and immediately processed. gDNA was extracted from 1 g of roots or 1 g of soil, using the PowerSoil DNA isolation kit (Mo Bio Laboratories, Carlsbad, CA, USA), according to the manufacturer’s instructions, with modifications. Each replicate sample was divided into four 250-mg subsamples in a separate bead tube supplied by the manufacturer with 500 ml extraction buffer. Tubes were agitated twice at 4.5 m s −1 using a cell disrupter (FastPrep FP120, BIO101, Savant). This agitation procedure optimizes yield of rhizoplane bacterial nucleic acids with minimal destruction of root tissue, thus minimizing plant-derived nucleic acids content in the samples. Following elution with solution C6, subsamples were pooled and purified and concentrated using the DNA clean & concentrator kit (Zymo Research, Irvine, CA, USA). DNA yield and quality were examined with an ND1000 spectrophotometer (NanoDrop Technologies, Wilmington, DE, USA), and agarose gel electrophoresis. Total RNA was extracted using a modification of the RNA PowerSoil Isolation Kit (Mo Bio Laboratories). Briefly, 1 g of roots or 4 g of soil were thawed on ice and 250 mg subsamples were immediately applied to the Mo Bio bead tubes. Total RNA was then extracted according to the manufacturer’s protocol with slight modifications. Then 10 μl ml −1 β-mercaptoethanol (Sigma-Aldrich, St Louis, MO, USA) were added into the bead solution. Following the addition of solution SR4, the incubation took place at room temperature for 40 min. After resuspension of RNA with solution SR7, subsamples of each replicate were pooled and then purified and concentrated using the RNA Clean & Concentrator kit (Zymo Research). Total nucleic acids were subjected to DNAse (Sigma-Aldrich) treatment. Approximate RNA concentrations and purity were determined using an ND1000 spectrophotometer (NanoDrop Technologies). In addition, complete removal of DNA was verified by PCR. Ribosomal RNA depletion and synthesis of ds-cDNA Ribosomal RNA (rRNA) constitutes the majority of total RNA species in transcriptomes and metatranscriptomes and challenges sequence-based analyses of mRNAs from microbial isolates and communities [33] . To reduce rRNA levels and amplify mRNA, the ExpressArt Bacterial mRNA Amplification Kit (AmpTec, Hamburg, Germany), was used. This kit selects against rRNA at the first strand cDNA synthesis stage, due to TRinucleotide primer, that binds selectively to the 3′ end of mRNA. The initial amount of total RNA used for amplification from root samples was 1,200 ng. Due to the inhibitory effect of carry-over soil contaminants, the amount of total RNA used for soil samples was 400 ng. Resulting amplified RNA (aRNA) amounts produced ranged between 13.26 and 18.27 μg for root samples and between 2.9 and 4.02 μg for soil samples. Total RNA quality and rRNA removal efficiency were evaluated using an Agilent 2100 Bioanalyzer (Agilent Technologies, Palo Alto, California, USA). Accordingly, the RNA Integrity Number was on average 6.13, and the removal of rRNA was above 90%. The resulting aRNA was converted into double-stranded complementary DNA (ds-cDNA) using the Micro dsDNA Synthesis Add-On Module (AmpTec). The starting amount of aRNA used for ds-cDNA synthesis was 5 μg from root samples and the total amount of aRNA from the soil samples (see above). Yields of ds-cDNA were estimated by NanoDrop ND1000 spectrophotometer and were on average 1.2 μg. Preparation of libraries and sequencing Genomic DNA extracted from soils and roots was processed for metagenomic sequencing using a Nextera dual-indexed DNA sample preparation kit, according to the manufacturer’s instructions (Illumina Inc., San Diego, CA, USA). Fifty nanograms of genomic DNA was used as input, and after processing and purification, library fragments of 400–800 bp in size were selected using a PippinPrep automated electrophoresis device (Sage Science, Beverly, MA, USA). Individual libraries were quantified using the KAPA library qPCR quantification kit for Illumina (KAPA Biosystems, Woburn, MA, USA), pooled in equimolar ratio, and purified again. The final library concentration was adjusted to 10 nM after a subsequent quantification reaction. Pooled libraries were prepared at the DNA Services (DNAS) Facility (University of Illinois at Chicago; UIC) and sequenced on an Illumina HiSeq2000 instrument (High-Throughput Sequencing and Genotyping Unit, University of Illinois at Urbana-Champaign; UIUC), with paired-end 100 base reads. In total, 410–527 million reads (combined forward and reverse reads) were recovered from each lane. Double-stranded complementary DNA, generated as described above, was prepared for metatranscriptome sequencing using the Nextera dual-indexed DNA sample preparation kit, as described above. DNA library fragments in the range of 150–350 bp were selected using the PippinPrep device, and equimolar pooling and library quantification were performed as described above. Pooled libraries were prepared at the DNAS facilities and were sequenced on an Illumina HiSeq2000 instrument (UIUC) with single-direction 100 base reads. In total we obtained 87.4 gigabase pairs (Gbp) of DNA in ten libraries: two libraries generated from cucumber soil, two libraries generated from wheat soil, three libraries from cucumber roots and three other libraries from wheat roots ( Supplementary Table 1 ). To generate an extensive catalogue of the soil and root microbiome, we first assembled the short Illumina reads into longer contigs, which could then be analysed and annotated by standard methods. We used Meta-velvet [34] pipeline based on velvet assembler [35] . We expected high variability between metagenomes of different niches, and therefore each niche was assembled independently: the four libraries of soil with a content of 34.9 Gbp were assembled separately and also the cucumber root niche containing 31.3 Gbp and wheat root niche containing 21.2 Gbp. The three assemblies of soil, cucumber root and wheat root resulted in 1,208,895 contigs with N50 of 217 bp, 1,228,889 contigs with N50 of 389 bp and 631,035 contigs with N50 214 bp, respectively. All contigs generated from the three assemblies were merged together. MetaGeneMark software [36] , [37] was used for detection of ORFs, using heuristic model for bacteria. To create a non-redundant set of ORF, we used the CD-HIT-EST software [38] using a similarity threshold of 95%. The ORFs generated served as our soil and root gene catalogue and includes 2,389,280 partial genes. To assign taxonomic and functional annotations, all detected ORFs were searched against the non-redundant NCBI protein database using the BLASTX algorithm [15] , [39] . Results were then uploaded to MEGAN software (version 4.70.4; ref. 40 ). The LCA algorithm was applied (parameters used with minimum bit-score of 70, minimum support of 5 and 30% top percent threshold) to compute the assignment of ORFs to specific taxa and for KEGG analysis. Following annotation, to generate taxonomic and functional count tables, each library was mapped to the gene catalogue with the Bowtie2 mapping software with default parameters [41] . The six metatranscriptome libraries generated (three from cucumber roots and three from wheat roots) produced 67.1 Gbp of sequence data, with high average quality scores between 35 and 36 ( Supplementary Table 1 ). Ribosomal RNA was filtered using SortMeRNA software [42] , which removed a large portion of the reads (82.8% on average, Supplementary Table 1 ). Each library was then mapped to the soil–rhizoplane gene catalogue using Bowtie2 mapping software and counts tables were generated. Between 22.6 and 34.8% of non-ribosomal reads were mapped to the gene catalogue ( Supplementary Table 1 ). The composition of reads within the wheat and cucumber rhizoplane metatranscriptomes is displayed in Supplementary Table 2 and Supplementary Fig. 4 . Data analysis All data analyses were done with R statistical software. To compare the taxonomic composition of root and soil bacterial communities, a bacterial counts table was parsed from the complete counts table. Then, counts were rarified to 5,000,000 reads per sample to eliminate bias related to differences in sample size, and binned into taxonomic groups, based on the BLASTX-MEGAN LCA annotation described above ( Supplementary Table 3 ). Principal component analysis was carried out with R package VEGAN (version 2.0–7). Variable (taxonomic groups) and factor correlations were calculated and ranked for the first and second principal components and ranked. The 10 variables with highest loadings were extracted and relative abundances of these groups were compared between soil and root (wheat and cucumber) communities, and between wheat roots and cucumber roots communities using nonparametric Mann–Whitney U -test ( P <0.05). For comparison of functional traits, the bacterial read counts table was binned into KEGG orthologous (KO) groups, based on BLASTX-MEGAN annotation. KOs with extremely few counts (three reads per million) were filtered out. To account for differences in library sizes, they were normalized by the trimmed means of M -values method [19] using the Bioconductor- edgeR package (version 3.2.4, ref. 20 ). Bray–Curtis similarities were pair-wise calculated between libraries and a heat map was drawn accordingly. Analysis of similarities was performed with the VEGAN package based on the Bray–Curtis distance matrix. Analysis of differential abundance between soil and root (wheat and cucumber) and between wheat root and cucumber root communities was conducted with edgeR package. A negative binomial model was applied, and differential abundance was tested, based on quantile-adjusted conditional maximum likelihood method. Differential abundance was considered significant under the conditions that the difference in abundance between communities was above twofold and FDR-adjusted P value was <0.01. In addition, differential abundance was assessed using the nonparametric SAMseq approach, which uses repeated permutations for assessment of the FDR. SAMseq [21] analysis was conducted with samr package. Analysis was performed using 1,000 permutations and 100 re-sampling of the data. Differential abundance was considered significant under the conditions that the difference in abundance between communities was above twofold and FDR-adjusted q value was <0.001. Comparison between metatranscriptome libraries of wheat roots and cucumber roots was done similarly, but the criteria for adjusted q value was amended to <0.05, due to lower number of samples. The list of all KOs found as differentially abundant between metagenomes or differentially expressed between metatranscriptomes and their overlap is presented in Supplementary Data 10 . To determine the specific composition of DA and DE KOs, the taxonomic affiliation of each related ORF was listed. Statistical composition based on relative contribution (%) of phyla and classes assigned to the KO groups were done using nonparametric Kruskal–Wallis analysis of variance ( P <0.05) followed by multiple comparisons with Bonferroni correction. Similarity percentage analysis [43] was performed using PAST software [44] to rank taxa according to their contribution to differences between taxonomic profiles down to the genus level. Accession codes: Sequences of soil and rhizoplane DNA and cDNA have been deposited in the NCBI Sequence Read Archive under BioProject accession number PRJNA208116 , biosample accession SAMN02202255 (experiments accessions: SRX310152, SRX310217 and SRX310215) and biosample accession SAMN02202255 (experiment accession SRX311002). How to cite this article: Ofek-Lalzar, M. et al. Niche and host-associated functional signatures of the root surface microbiome. Nat. Commun. 5:4950 doi: 10.1038/ncomms5950 (2014).